Featural and temporal attention selectively enhance task-appropriate representations in human primary visual cortex Our perceptions are often shaped by focusing our attention towards specific features or periods of time irrespective of location. Here we explore the physiological bases of these non-spatial forms of attention by imaging brain activity while subjects perform a challenging change-detection task. The task employs a continuously varying visual stimulus that, for any moment in time, selectively activates functionally distinct subpopulations of primary visual cortex (V1) neurons. When subjects are cued to the timing and nature of the change, the mapping of orientation preference across V1 systematically shifts towards the cued stimulus just prior to its appearance. A simple linear model can explain this shift: attentional changes are selectively targeted towards neural subpopulations, representing the attended feature at the times the feature was anticipated. Our results suggest that featural attention is mediated by a linear change in the responses of task-appropriate neurons across cortex during appropriate periods of time. A defining feature of visual attention is its flexibility. Subjects may selectively attend to locations, objects, periods of time and visual features to enhance their perceptual capabilities [1] , [2] , [3] , [4] . Of these, the selection according to location (spatial attention) is the most studied. Numerous studies have demonstrated that when subjects covertly attend to a location, the sensory responses of neurons representing this location are enhanced throughout the visual hierarchy [5] , [6] . Studies of single neurons in monkey visual cortex suggest that non-spatial attention is similarly targeted, such that attention preferentially enhances neurons selective for an attended feature [7] and attentional modulations are strongest during times that the animal is maximally focused [8] . These attentional modulations may be divided into two broad categories: linear, gain-like increases in a neural firing [9] ; and more complex non-linear modulations. While a variety of non-linear effects have been reported [10] , [11] , [12] , similar gain modulations have been observed in spatial [6] , [13] and featural [14] attention studies. Moreover, computational modelling suggests that some non-linear effects may actually arise from simple gain processes [15] . These findings lead us to hypothesize the existence of a single common mechanism for visual attention: while attending to a stimulus, simple but computationally powerful [16] gain modulations are targeted to the neurons and times most appropriate for the task at hand. Testing this theory requires the ability to systematically map the representation of a visual feature representation across an entire visual area to first identify the neural subpopulation best matched to the task and then measure how responses within that subpopulation change with attention and over time. To this end, the encoding of stimulus orientation within primary visual cortex (V1) is ideal. Within V1, a single cortical column contains neurons tuned towards a common orientation [17] , and recently developed functional magnetic resonance imaging (fMRI) techniques are capable of measuring orientation tuning at columnar resolutions [18] . Moreover, orientation tuning can be observed even in voxels, which are larger than a cortical column [19] . Such tuning offers an opportunity, for the first time, to map a non-spatial visual representation within a single cortical area and to study how that map is dynamically changed with attention. To address how representations of visual information are altered by non-spatial attention, we therefore imaged V1 using ultra-high field fMRI (7 T) while subjects performed a periodic non-spatial attention task [19] , [20] . We discovered that both orientation tuning and attentional modulations of that tuning, are present within individual voxels. Both the orientation preferences and the response timing of voxels systematically shift towards the featural and temporal foci of attention. These shifts can be explained by a model in which featural and temporal attention cause linear changes in activity preferentially directed during behaviourally appropriate times to neurons with appropriate feature selectively. Our results suggest that representations at the earliest stages of visual processing can be profoundly altered by cognitive influences and that all forms of attention may act by common mechanisms to selectively enhance behaviourally relevant sensory representations throughout cerebral cortex. Attention biases single-voxel orientation tuning Human subjects ( n =9, 7 male) participated in a visual change-detection task. Over a 5 min trial, subjects viewed a continuously rotating (20 s period, 15 rotations per trial), full field, counter-phasing Gabor grating and quickly responded by button press when the spatial frequency (SF) of the stimulus briefly (50–83 ms) doubled ( Fig. 1a ). This task was demanding (60% hit/17% false alarm rate) and required the subjects’ continuous vigilance. To manipulate attention, there was a non-uniform probability of SF changes occurring; subjects were cued prior to each trial to the range of orientations at which changes were most likely. Two types of attention trials were presented: one in which changes were more likely around 45° (Attend 45° (A45)) and the other at 135° (Attend 135° (A135)). Subjects responded quickly to expected SF changes and suffered a small but significant penalty in reaction time to unexpected SF changes ( Fig. 1c , 15–22 ms, Rayleigh test, P <0.01). The range of orientations associated with quick reaction times (95°, Fig. 1c ) was nearly identical to the range of orientations at which changes were most likely (87°). However, during a control condition in which change probability was constant over all orientations (No-Cue), subjects were uniformly quick to identify the changes with no behavioural bias in favour of one orientation. The uniformly fast No-Cue reaction times suggest that our attentional manipulation behaviourally encouraged subjects to ignore the stimulus during periods when the SF change was unlikely. During an alternative control in which the stimulus was fixed to vertical and did not rotate but change probabilities still varied (No-Rotate), subjects still showed the penalty towards unexpected changes (21 ms). We concluded that subjects selectively attended to the stimulus when changes were likely, although with an anticipatory advance between peak attentional effect and peak stimulus probability. 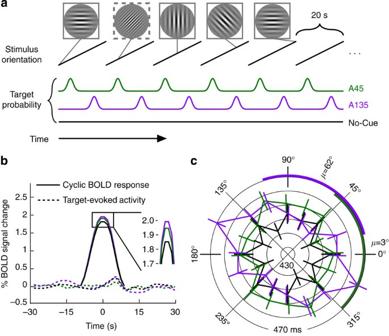Figure 1: Selective attention in a change-detection task. (a) Human subjects viewed a full-field, continuously rotating Gabor and responded by button press when the spatial frequency of the stimulus briefly changed (dashed outline). During attention conditions, these target events were more likely to occur at a single orientation (green, A45; violet, A135). Prior to each trial, a static grating indicated to the subject the orientation about which targets are likely to occur. In one control condition, the target probability is static over time (No-Cue, black). (b) Mean event-related response to stimulus rotation (aligned to preferred phase, solid) and to target events (dashed, aligned to individual target events per condition) averaged across all voxels with significant orientation selectivity. The response to individual target events was negligible, but removed via linear regression in all future analyses. The mean global response increased with attention. (c) Reaction time, indicated by radius, is fastest prior to the cued orientation when subjects anticipate target events.μ, orientation with the fastest mean response during each Attend condition; coloured arc, full-width at half-maximum (FWHM) range of fastest reaction times (A45 FWHM 98° and A135 FWHM 92°). Figure 1: Selective attention in a change-detection task. ( a ) Human subjects viewed a full-field, continuously rotating Gabor and responded by button press when the spatial frequency of the stimulus briefly changed (dashed outline). During attention conditions, these target events were more likely to occur at a single orientation (green, A45; violet, A135). Prior to each trial, a static grating indicated to the subject the orientation about which targets are likely to occur. In one control condition, the target probability is static over time (No-Cue, black). ( b ) Mean event-related response to stimulus rotation (aligned to preferred phase, solid) and to target events (dashed, aligned to individual target events per condition) averaged across all voxels with significant orientation selectivity. The response to individual target events was negligible, but removed via linear regression in all future analyses. The mean global response increased with attention. ( c ) Reaction time, indicated by radius, is fastest prior to the cued orientation when subjects anticipate target events. μ , orientation with the fastest mean response during each Attend condition; coloured arc, full-width at half-maximum (FWHM) range of fastest reaction times (A45 FWHM 98° and A135 FWHM 92°). Full size image To study how such selective attention altered representations in early visual cortex, we obtained ultra-high field, high resolution blood-oxygen level dependent (BOLD) functional images from a large volume of occipital cortex (7 T, GE sequence, 690–1,050 cm 3 image volume, 1.5 × 1.5 × 1.5 mm voxel size and TE/TR 20/1,500 ms), while subjects performed the task. We discarded data from one subject due to substantial motion artifacts. For the remaining eight subjects, we explored response tuning for individual voxels within a V1 region-of-interest (ROI) that was defined on the basis of anatomy and retinotopy. During all trials, the stimulus rotated at the same constant rate ( Fig. 1a ). Thus, for orientation-selective voxels, we would expect that the BOLD response would show modulations over time at this frequency [18] . The phase of such modulation could reflect the preferred orientation of the voxel, while the amplitude would reflect its orientation selectivity. Alternatively, a voxel with a 20-s periodic response could also be temporally selective and show activity during a specific time point in the stimulus cycle without any orientation-specific visual processing. Thus the peak of a voxel’s cyclic response could correspond to a preferred orientation or to a preferred time; we will use the term ‘preferred phase’ to avoid the assumption that all cyclic activity is necessarily orientation selective. A major goal of our analysis will be to determine the relative contributions of orientation and temporal attention within V1 (see below), but to study such contributions we must first establish that voxels are all modulated according to the orientation/temporal rhythm. In all runs from all subjects, we observed single voxels with significant tuning to our stimulus as evidenced by BOLD modulation at the orientation frequency. An example voxel is shown in Fig. 2a . To quantify this selectivity, we computed the likelihood that each voxel’s maximum and minimum BOLD activity could be used to distinguish between the voxel’s preferred and anti-preferred stimulus phase. This is analogous to a classical decoding framework, only adapted for our continuous paradigm (see Methods). We found that a substantial proportion of individual voxels could distinguish between orthogonal orientations with >95% accuracy ( Fig. 2b ). This is in sharp contrast to most fMRI studies of human V1 (refs 21 , 22 ), which have been unable to find individual voxels with significant decoding performance. Moreover, the performance of many individual voxels in our sample exceeds the overall performance reported in previous studies (≈70%) when thousands of V1 voxels were analyzed together. 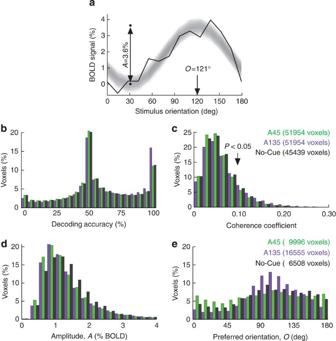Figure 2: Orientation-selectivity in single V1 voxels. (a) Fourier and regression analysis (see Methods) provides the amplitude (A) and peak (O) of each voxel’s orientation tuning curve. Peaks are offset to account for the haemodynamic lag between stimulus presentation and BOLD response. Shaded region shows a confidence interval of the fitted sine wave for this example voxel. Orientation-selectivity metrics for this voxel: coherence coefficient=0.2131 (P=1.7 × 10−5), decoding accuracy≈100%. (b) Many individual voxels accurately discriminate between their preferred and anti-preferred orientations (mode at 50% represents chance performance). (c) Many voxels have significant coherence at the signal frequency. Coherence coefficient of 0.0984 (arrow) is the threshold for statistical significance. (b,c) include all V1 voxels. (d) Among orientation-selective voxels, attention recruited weakly orientation-selective voxels. (e) Among orientation-selective voxels, the distribution of preferred orientations is biased towards the attended orientation. Figure 2: Orientation-selectivity in single V1 voxels. ( a ) Fourier and regression analysis (see Methods) provides the amplitude (A) and peak (O) of each voxel’s orientation tuning curve. Peaks are offset to account for the haemodynamic lag between stimulus presentation and BOLD response. Shaded region shows a confidence interval of the fitted sine wave for this example voxel. Orientation-selectivity metrics for this voxel: coherence coefficient=0.2131 ( P =1.7 × 10 −5 ), decoding accuracy≈100%. ( b ) Many individual voxels accurately discriminate between their preferred and anti-preferred orientations (mode at 50% represents chance performance). ( c ) Many voxels have significant coherence at the signal frequency. Coherence coefficient of 0.0984 (arrow) is the threshold for statistical significance. ( b , c ) include all V1 voxels. ( d ) Among orientation-selective voxels, attention recruited weakly orientation-selective voxels. ( e ) Among orientation-selective voxels, the distribution of preferred orientations is biased towards the attended orientation. Full size image A notable exception exists for studies, utilizing ultra-high resolution over a restricted volume of V1 (less than and equal to four slices) [18] , [19] , which have demonstrated orientation-selective responses from single V1 voxels. To enable comparison to these reports, we also computed a coherence coefficient (CC) to estimate the degree to which each voxel is entrained to the stimulus frequency. While Sun et al . [19] reported 35.3% of voxels were significantly coherent with the stimulus, we only found such coherence in 15.6% of voxels at baseline ( Fig. 2c ). Thus, while our imaging parameters allowed for the greatest sensitivity to orientation tuning that has yet been reported for high-volume imaging using isometric voxels, these parameters did not afford a functional resolution equal to that of dedicated ultra-high resolution/low-volume methodologies. To restrict the remainder of our analyses to voxels which exhibited a significant degree of tuning, we utilized regression analysis to make a binary decision, for each voxel, as to whether its response was significantly entrained by the stimulus. In comparison to the coherence analysis above, this regression analysis was performed without detrending or other manipulation of the frequency content within each voxel. Across all subjects, we found that 14.3% of voxels exhibited such significant tuning (regression F -test, restricted to 5% false positives) during No-Cue conditions ( Fig. 3a ). 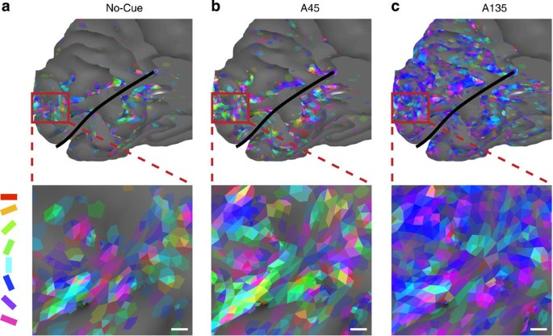Figure 3: Attention biases the orientation preference map. (a) Preferred orientation from one subject, coded by colour and measured during No-Cue task, plotted on a medial view of occipital cortex. Inset is a flattened representation of the occipital pole. Greater colour saturation indicates a higher certainty in preference estimate. Orientation selectivity was greatest along gyri, likely due to the use of a surface coil. (white scale bar, 2 mm; black line, calcarine sulcus). (b,c) Asa, with orientation preference measured during the attention conditions. Attention increased the extent of orientation-selective activity across the occipital cortex (top) and biased population orientation preferences at the hyper-columnar scale (bottom). Figure 3: Attention biases the orientation preference map. ( a ) Preferred orientation from one subject, coded by colour and measured during No-Cue task, plotted on a medial view of occipital cortex. Inset is a flattened representation of the occipital pole. Greater colour saturation indicates a higher certainty in preference estimate. Orientation selectivity was greatest along gyri, likely due to the use of a surface coil. (white scale bar, 2 mm; black line, calcarine sulcus). ( b , c ) As a , with orientation preference measured during the attention conditions. Attention increased the extent of orientation-selective activity across the occipital cortex (top) and biased population orientation preferences at the hyper-columnar scale (bottom). Full size image We then repeated these analyses for our Attend trials. We found that attention to a cued orientation increased the median decoding accuracy and CC among all V1 voxels, as well as the prevalence of selective voxels in all subjects: 19.2% (A45, Fig. 3a ) to 31.9% (A135, Fig. 3b ) of voxels collected during attend conditions were significantly correlated to the stimulus. This recruitment is consistent with known neurophysiology: attention to one orientation causes orientation tuning to emerge in otherwise non-orientation-selective neurons in V4 (ref. 6 ), and an attention-mediated increase in activity should cause weakly selective voxels to show a more robust and detectable modulation. The stronger attentional effects of the A135 condition, as compared with the A45 condition, likely reflect the predominance of vertically tuned voxels in our sample ( Fig. 2e ) and the behavioural ( Fig. 1c ) evidence, suggesting that subjects anticipated likely changes and accordingly increased their attention prematurely (that is, during the presentation of vertical lines during the A135 condition). Attention increased the mean amplitude of cyclic activity across V1/V2 ( Fig. 1b ), though increases in the number of both low- and high-amplitude voxels are observed (tails of the distribution in Fig. 2d ). In addition to increasing stimulus selectivity, attention powerfully biased voxels’ baseline (No-Cue) phase preferences. The distribution of phase preferences spanned the entire range of orientations, but was non-uniform in all conditions. During the No-Cue condition we saw an innate bias towards post-vertical phases (90°–135°), whereas preferred phases were biased from the No-Cue distribution towards the cue during the Attend conditions ( Figs 2e and 3 ). Thus attention both increased phase selectivity and shifted phase preferences towards the cued orientation. If these were the only task-related changes occurring within the brain, we would expect that such changes would decrease subjects’ reaction times, as information about the stimulus is accumulated faster. We, however, observed the opposite: the cue instead increased average reaction times across all stimuli ( Fig. 1c ). This suggests that task-related non-specific changes, such as motor preparation or vigilance, which are likely to present in numerous areas other than V1, significantly contributed to the overall behaviour. Such non-specific behaviour effects open up the possibility that V1 changes might simply reflect overall task parameters, rather than task-related changes in stimulus representation associated with attention. To examine whether such changes in BOLD response phase may occur irrespective of the actual stimulus presented, we applied identical analysis techniques for data from No-Rotate trials. During this condition, only 0.5% of voxels were cyclically active and no single voxel cycled during two different scans. Thus the temporal pattern of SF changes was not sufficient to evoke V1 activity; the cyclic activity we observed is a result of cyclic visual stimulation. Moreover, cyclic changes in BOLD response cannot be explained by the biased distribution of SF changes, because such changes failed to evoke a measurable BOLD response ( Fig. 1b ) and would therefore be unable to skew the BOLD signal at the paradigm’s fundamental frequency. Thus the observed changes in orientation tuning were due to a top-down modulation of innate orientation-selective responses in V1 and do not reflect differences in stimulation between the attention runs. Because we observed voxels with tuning preferences across the entire 180° range for all three conditions, we could examine whether attention modulations were selectively directed to neural populations appropriate to the particular attention condition. We first identified those voxels which had significant phase selectivity during both the No-Cue and attention conditions (voxels that ‘Stay-On’ with attention, n =7,969). During attention trials, Stay-On voxels on average reached peak activity earlier, such that they either had a more clock-wise preferred orientation (5.40°) or had a more rapid haemodynamic response (0.60 s, Upton’s angular mean test, n =7,969, P <10 −10 ). However, this tuning advance was a function of voxel phase preference: when a single orientation was cued, the response of voxels with a preference at or after the cue was shifted towards the cue ( Fig. 4a,b ). As expected, the cue-selectivity of attention effects was largely orthogonal between the A45 and A135 conditions (as was observed with subject reaction times). By directly comparing voxels that were selective during both attention conditions ( Fig. 4c ), we found that 36.3% of voxels had a significant difference in orientation preference (likelihood estimation, 356–716 Degree of Freedom (DOF), q FDR <0.01). 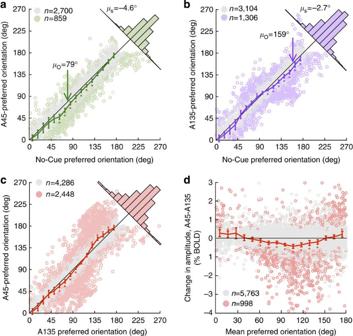Figure 4: Attention selectively advances and amplifies orientation tuning curves. (a) Voxels with an orientation preference near 79° respond sooner (have a less positive orientation preference) during A45 condition. Error bars show 99.9% confidence intervals of the mean. Note that 270° is equivalent to 90°. Inset histogram shows distribution of tuning preference shifts as distance from the identity line. (black line, identity line;μO, centre of range with significant tuning advance;μS, mean tuning curve advance over all voxels). Colour indicates individual voxels that are at a significant (qFDR<0.01, likelihood estimation) distance from the identity line. (b) Asa, showing an orthogonally distributed tuning curve advance during A135. (c) Direct comparison between A45 and A135 conditions reveals a strong and orthogonal relationship between preferred orientation and changes in tuning preference. (d) Asc, comparing tuning amplitude between A45 and A135. Amplitude increases for voxels with preference prior to the attended orientation (‘*’ indicates significant change, von Mises (a–c) ort-test (d), variable DOF,P<0.001). Figure 4: Attention selectively advances and amplifies orientation tuning curves. ( a ) Voxels with an orientation preference near 79° respond sooner (have a less positive orientation preference) during A45 condition. Error bars show 99.9% confidence intervals of the mean. Note that 270° is equivalent to 90°. Inset histogram shows distribution of tuning preference shifts as distance from the identity line. (black line, identity line; μ O , centre of range with significant tuning advance; μ S , mean tuning curve advance over all voxels). Colour indicates individual voxels that are at a significant ( q FDR <0.01, likelihood estimation) distance from the identity line. ( b ) As a , showing an orthogonally distributed tuning curve advance during A135. ( c ) Direct comparison between A45 and A135 conditions reveals a strong and orthogonal relationship between preferred orientation and changes in tuning preference. ( d ) As c , comparing tuning amplitude between A45 and A135. Amplitude increases for voxels with preference prior to the attended orientation (‘*’ indicates significant change, von Mises ( a – c ) or t -test ( d ), variable DOF, P <0.001). Full size image We also explored the effect of attention on the amplitude of single-voxel tuning curves. Across all voxels, the cue increased tuning amplitude by 0.034±0.015% BOLD (95% confidence interval, t -test, 7,968 DOF, P =0.041). This increase was less robust and only reached significance in 14.7% (likelihood estimation, 356–716 DOF, q FDR <0.01) of Stay-On voxels ( Fig. 4d ). But, as with phase preference, these effects were selective and depended on preferred phase: attention to a cue increased the response amplitude of voxels whose preference aligned with the period of maximal behaviour effect (before the cue). Because our task utilized a full-field stimulus, subjects should gain no benefit from applying spatial attentional strategies. However, because spatial attention was not explicitly controlled, it is possible that subjects focused their attention spatially and that focus differed between our A45 and A135 conditions. If this were true, one would expect attentional modulations would vary significantly across the visual field and differentially between the two attention conditions. We therefore examined whether phase preferences of individual voxels, and attentional modulation of those preferences, varied according to retinotopic position. Consistent with previous reports [23] , we found a significant correlation between preferred phase and retinotopic polar angle (angle–angle correlation, r 2 : 0.07–0.13) at parafoveal eccentricities. However, our attentional effects were uniform across the visual field: retinotopy was uncorrelated with the changes in preference or amplitude seen in our attention trials (regression analysis, Supplementary Fig. 1 ). This confirmed that the modulations we report were targeted to individual V1 voxels solely as a function of their featural tuning. Attention linearly increases BOLD activity over all of V1 While these results establish that appropriate neuronal populations in human V1 are preferentially modulated by attention, they do not speak about the nature of this modulation. Numerous imaging and electrophysiological studies suggest that spatial attention has a simple linear effect on responses [9] . In these studies, attention either multiplies (‘gain’ effect) or increases (‘additive’ effect) responses across a range of stimulus conditions. In the context of neurons tuned to a particular parameter, such as orientation in early visual areas, the model predicts that attention will increase orientation tuning curve amplitudes without any changes in preference. When a neuronal population with a variety of preferred orientations is sampled, such as individual voxels in our study, this model permits that the overall orientation tuning of the sampled population may change in preference, in accordance with our observations. However, because previous studies have been unable to reveal and map functional preferences other than retinotopy in the human it has not been possible to examine linear non-spatial attention models in humans. By contrast, our ability to observe significant tuning in a large number of voxels within V1 enables us to systematically compare tuning curves across our attention conditions. To do this, we first grouped Stay-On voxels according to their preferred orientation relative to the attended orientation, combining A45 and A135 into a single normalized Attend data set. We tested whether a linear model could explain how the mean orientation tuning curves (computed over all voxels, grouped by orientation preference into 13 bins and overall 13 sampled time points) changed with attention ( Fig. 5 ). Across all orientation preferences and all points of time, a simple linear regression provided a good explanation of the effects of attention on V1 activity. Having demonstrated that orientation tuning curves between two conditions were linearly related, we wanted to further determine whether the effects of attention might also be well-described as linear modulations within the voxels that gained or lost tuning with attention. Thus we repeated this analysis using voxels that only showed significant phase selectivity during the Attend conditions (voxels that ‘Turn-On’ with attention, n =13,876 across both attention conditions) or only during the No-Cue condition (‘Turn-Off’, 5,047 voxels). Even in the absence of well-defined single-voxel tuning curves, we found that the average BOLD signals between the Attend and No-Cue conditions were also well-described by a simple linear model ( Fig. 5 ). Across all voxel groups, we also observed positive linear correlation coefficients between the single-voxel tuning curves estimated from No-Cue and Attend data, even when these tuning curves were not significantly tuned (median correlation coefficient: Stay-On 0.72, Turn-On 0.36 and Turn-Off 0.31; Supplementary Fig. 2 ). 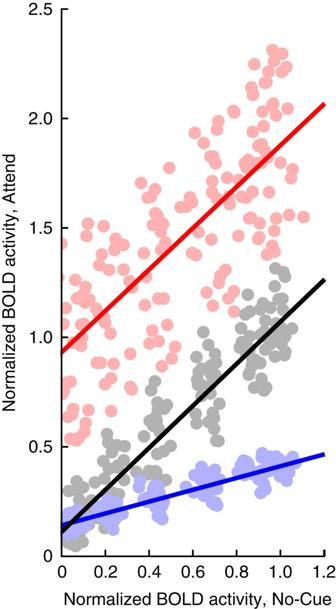Figure 5: Attentional modulations are linear over V1. Normalized activity (see Methods) during No-Cue and Attend conditions is highly similar in Stay-On voxels (grey). Each point represents the mean normalized activity of all voxels with a set range of phase preferences over a single sample interval; preference and time are sampled to 13 points each, providing 169 data points. The effect of attention over all points is well-described by a linear fit (R2=0.92, slope 0.96,y-intercept 0.11). Changes in tuning curves observed in Turn-On (red) and Turn-Off (blue) voxels are also relatively well-described by linear functions (Turn-On:R2=0.61, slope 0.95, y-intercept 0.93; Turn-Off:R2=0.86, slope 0.27,y-intercept 0.14). Figure 5: Attentional modulations are linear over V1. Normalized activity (see Methods) during No-Cue and Attend conditions is highly similar in Stay-On voxels (grey). Each point represents the mean normalized activity of all voxels with a set range of phase preferences over a single sample interval; preference and time are sampled to 13 points each, providing 169 data points. The effect of attention over all points is well-described by a linear fit ( R 2 =0.92, slope 0.96, y -intercept 0.11). Changes in tuning curves observed in Turn-On (red) and Turn-Off (blue) voxels are also relatively well-described by linear functions (Turn-On: R 2 =0.61, slope 0.95, y-intercept 0.93; Turn-Off: R 2 =0.86, slope 0.27, y -intercept 0.14). Full size image Although our ultimate goal is to determine whether attentional modulations act with specificity over features and time, we used these linear fits both within single voxels and over the entire data set to justify the assumption that any featurally or temporally specific effects should be linear as well. This simplifying assumption enabled us to utilize a two-dimensional model to disambiguate between temporal and featural attentional mechanisms. Dissociation of featural and temporal attention mechanisms The possibility that attention is modulated both over time and feature preference presents a potential challenge, because both featural and temporal modulations may enhance neural activity in a subset of voxels. Moreover, our periodic stimulus naturally confounds orientation and time at the level of single voxels. However, we can use the fact that the full range of orientation preferences exist among sample voxels to distinguish the two types of attention. This is because feature-specific modulations should cause modulation among voxels of an appropriate orientation selectivity but irrespective of time. Similarly, time-specific modulation should cause modulations in all sampled voxels irrespective of their feature preference. Thus, a model that simultaneously incorporates both types of modulations can be used to quantify the effect that can be attributed to each type of attention. To evaluate such a model, we computed a population activity surface in which normalized BOLD responses from Stay-On voxels in the No-Cue condition are binned according to stimulus time relative to the attended time and by the preferred orientation of the voxel relative to the attended orientation ( Fig. 6a ). We then constructed a similar response surface for the same voxels in the Attend conditions ( Fig. 6c ), using the same grouping as used for the No-Cue surface. Examination of this response surface reveals that maximal responses in the Attend case are not present at the cued orientation/time, but rather slightly precede the cue both in time and in preferred orientation. The anticipation is consistent with our behavioural ( Fig. 1c ) and amplitude ( Fig. 4d ) data, in which maximal effects precede the cued orientation. 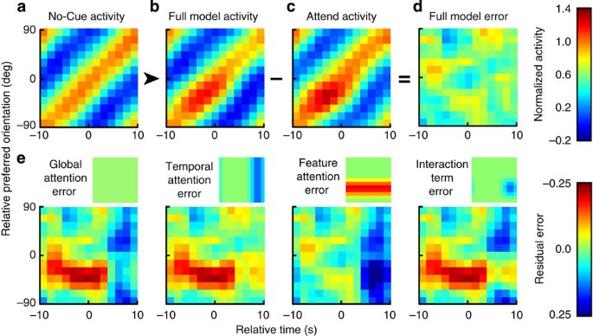Figure 6: A combination of featural and temporal mechanisms is required to explain attentional changes in orientation tuning. (a) Normalized BOLD activity during No-Cue condition, averaged across all subjects and retinotopic locations, for the Stay-on voxel group. Each row represents the mean tuning curve (response over the stimulus cycle) for voxels that share a common orientation preference relative to the cue. Orientation and time are given relative to the cue, which occurs at 0°/0 s. (b) The No-Cue activity surface is enhanced by a linear transformation and phase advance (0.6 s) to most closely approximate the corresponding Attend activity surface (c) defined from the same voxels with the same scaling. (d) The residual difference between the observed (c) and predicted (b) Attend activity is small (R2=0.99,Radj2=0.82 after removing variance due to global effects (see Methods)). The Bayesian information criterion is used to compare this full model with simpler submodels to determine which mechanisms of attention are most consistent with these data. (e) The model inbis generated from the sum of four different attentional mechanisms (small images): a global term which modulates all data points equally, featural and temporal terms which act purely as a function of either the feature (row) or time (column) dimension, and an interaction term which acts with both featural and temporal specificity. All terms may incorporate both a multiplicative and additive component (that is, are linear functions of the formy=mx+b, see Methods); however only additive effects are shown in this and inFig. 7, as multiplicative modulations were not statistically justified. Each attentional mechanism alone is insufficient to explain the effects of attention, as shown by the patterned error surfaces produced when only one mechanism is modelled. Figure 6: A combination of featural and temporal mechanisms is required to explain attentional changes in orientation tuning. ( a ) Normalized BOLD activity during No-Cue condition, averaged across all subjects and retinotopic locations, for the Stay-on voxel group. Each row represents the mean tuning curve (response over the stimulus cycle) for voxels that share a common orientation preference relative to the cue. Orientation and time are given relative to the cue, which occurs at 0°/0 s. ( b ) The No-Cue activity surface is enhanced by a linear transformation and phase advance (0.6 s) to most closely approximate the corresponding Attend activity surface ( c ) defined from the same voxels with the same scaling. ( d ) The residual difference between the observed ( c ) and predicted ( b ) Attend activity is small ( R 2 =0.99, R adj 2 =0.82 after removing variance due to global effects (see Methods)). The Bayesian information criterion is used to compare this full model with simpler submodels to determine which mechanisms of attention are most consistent with these data. ( e ) The model in b is generated from the sum of four different attentional mechanisms (small images): a global term which modulates all data points equally, featural and temporal terms which act purely as a function of either the feature (row) or time (column) dimension, and an interaction term which acts with both featural and temporal specificity. All terms may incorporate both a multiplicative and additive component (that is, are linear functions of the form y = mx + b , see Methods); however only additive effects are shown in this and in Fig. 7 , as multiplicative modulations were not statistically justified. Each attentional mechanism alone is insufficient to explain the effects of attention, as shown by the patterned error surfaces produced when only one mechanism is modelled. Full size image Having constructed these two response surfaces, we then tested whether global, temporally specific and featurally specific modulations could explain the effects of attention. Consistent with the global effect of attention seen across all voxels ( Fig. 5 ), we first modelled our attention data by invoking a non-specific modulation ( Fig. 6e ) that has uniform effects across all neurons and time. In this model, we found a systematic pattern of error along the diagonal of the surface. To account for these errors, we introduced a global response advance to the Attend responses of our model. Such a term may represent a systematic decrease in the haemodynamic response latency of V1/V2 during Attend conditions or a selective increase of the leading tail of all orientation tuning curves. This is consistent with our previous observation of a change in orientation preference across all voxels ( Fig. 4 ). Once this global phase shift was introduced, along with global attentional effects, we found a pattern of errors consistent with specific and directed allocations of spatial and featural attention. Accordingly, we then found the specific featural, and temporal attention functions, that when applied over the rows (featural dimension) and columns (temporal dimension) of the No-Cue activity surface best explains the Attend surface. Our full model contains four attentional mechanisms: a global modulation; additive featural and temporal modulations; and the feature-time interaction. Notably, these mechanisms are consistent with previous reports: attention is typically observed to be an additive/constant modulation in BOLD studies [24] and human visually evoked potentials suggest that featural and temporal attention may act synergistically [25] . The parameters of this model are shown in Fig. 7 , and cross-validated in Supplementary Fig. 3 . While the mode of the feature attention facilitation anticipates the cue by 32°, its width averaged across all voxels (80°) is comparable to the width of orientations over which behavioural events were most likely to occur (87°) and over which behavioural responses were most altered (95°, Fig. 1d ). Conversely, we found a temporal suppression across all voxels after the cued time. Thus our feature and temporal attention functions are well-matched to the behavioural manipulation. The interaction term is negative and compensatory to the feature attention term, acting to limit the feature-based modulation to only the most relevant points of time ( Fig. 7d ). 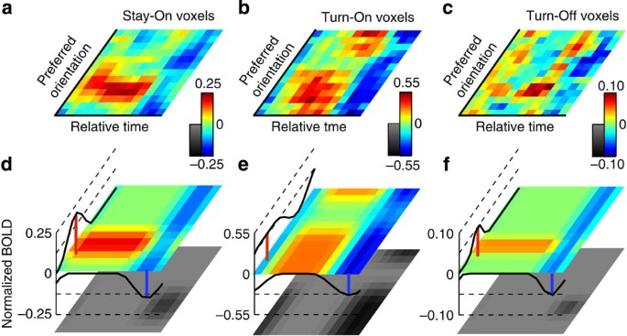Figure 7: Attention model parameters from three separate groups of voxels are nearly identical. The optimal model (lowest BIC) is comprised of three attentional mechanisms: a feature-specific additive enhancement, a time-specific subtractive inhibition and an inhibitory interaction term, which gates the feature-attention to the relevant period of time. (a) The empirical attention surface generated from Stay-On (SO) voxels, computed as the difference between the Attend and No-Cue activity surfaces. Variance that is explained by global changes in activity over all voxels (the trend line inFig. 5) has been removed. The middle of this surface represents the cued orientation/time. (b,c) Asa, showing the attention surfaces generated from Turn-On (ON) and Turn-Off (OFF) voxels. All surfaces show an increase in activity within voxels that prefer an orientation just prior to the cue, and all surfaces show a global suppression after the stimulus passes the cued orientation. (d) The best-fitting model surface for the SO voxel attention surface. Curves along the left and bottom sides show the modelled featurally and temporally specific modulations, while the black-and-white surface shows the feature-time interaction term (always suppressive). The sum of all three attentional mechanisms provides the coloured model surface. (e,f) Asd, showing models derived for the ON and OFF voxels. All three models approximate their respective attention surfaces well (Radj,SO2=0.82,Radj,ON2=0.80,Radj,OFF2=0.44), and all three models agree as to when and where V1 attentional modulations are found (featural attention peaks: SO −32°, ON −52° and OFF −34°; featural attention widths: SO 51°, ON 115° and OFF 30°; temporal attention peaks: SO 63°, ON 71° and OFF 66°; temporal attention widths: SO 47°, ON 64° and OFF 36°). Figure 7: Attention model parameters from three separate groups of voxels are nearly identical. The optimal model (lowest BIC) is comprised of three attentional mechanisms: a feature-specific additive enhancement, a time-specific subtractive inhibition and an inhibitory interaction term, which gates the feature-attention to the relevant period of time. ( a ) The empirical attention surface generated from Stay-On (SO) voxels, computed as the difference between the Attend and No-Cue activity surfaces. Variance that is explained by global changes in activity over all voxels (the trend line in Fig. 5 ) has been removed. The middle of this surface represents the cued orientation/time. ( b , c ) As a , showing the attention surfaces generated from Turn-On (ON) and Turn-Off (OFF) voxels. All surfaces show an increase in activity within voxels that prefer an orientation just prior to the cue, and all surfaces show a global suppression after the stimulus passes the cued orientation. ( d ) The best-fitting model surface for the SO voxel attention surface. Curves along the left and bottom sides show the modelled featurally and temporally specific modulations, while the black-and-white surface shows the feature-time interaction term (always suppressive). The sum of all three attentional mechanisms provides the coloured model surface. ( e , f ) As d , showing models derived for the ON and OFF voxels. All three models approximate their respective attention surfaces well ( R adj,SO 2 =0.82, R adj,ON 2 =0.80, R adj,OFF 2 =0.44), and all three models agree as to when and where V1 attentional modulations are found (featural attention peaks: SO −32°, ON −52° and OFF −34°; featural attention widths: SO 51°, ON 115° and OFF 30°; temporal attention peaks: SO 63°, ON 71° and OFF 66°; temporal attention widths: SO 47°, ON 64° and OFF 36°). Full size image To further test the model, we examined whether attentional changes in a tuning parameter that was not explicitly fit, namely the selectivity of individual voxels, were also accurately predicted. Although there was considerable variance in this tuning width data, on average, a clear bimodal pattern of width changes as a function of phase preference was present in both the A45 and A135 data ( Supplementary Fig. 4 ). Moreover, both the shape and amplitude of this bimodal pattern of tuning width changes was largely replicated in our attentional model. To further validate these findings, we independently repeated the modelling analysis on the Turn-On and Turn-Off voxel subgroups. As a group, these attentional surfaces had greater noise and greater model errors. However, the featural, temporal and feature-time interaction parameter estimates derived from both Turn-On and Turn-Off voxels ( Fig. 7e,f ) are well-correlated with those estimates obtained from Stay-On voxels. In all voxel subgroups, featural attention was characterized by a facilitation, which was maximally directed to voxels whose preference preceded the cued orientation but restricted in time by a negative interaction term, and temporal attention was characterized by a suppression that was maximal after the cued orientation was presented. We concluded that across all subjects and all voxels, the major mechanisms of attention were an increase in activity that is targeted to voxels with an appropriate feature preference and a suppressive effect gated as a function of the temporal rhythm of the task. We have shown that population activity in V1 is selectively enhanced during non-spatial forms of visual attention. While V1 cortical columns are tuned across several dimensions, the most prominent are tuning to retinotopic location and to stimulus orientation (spatial and featural tuning). Just as spatial attention enhances activity in populations that are tuned towards the attended region of space regardless of their feature tuning, we found that attention to a visual feature selectively enhances neural populations tuned towards that feature irrespective of spatial tuning. Considering the findings that modality-specific attention enhances stimulus selectivity in primary auditory [26] and somatosensory cortices [27] , we interpret our data as consistent with the overarching hypothesis that attention selectively targets the neural sub-populations within the earliest levels of sensory processing that are best suited for a task irrespective of modality. We were able to simultaneously measure featural tuning and attentional modulations across large portions of V1. The sensitivity of the BOLD signal to attentional modulations is well-known [28] , [29] even within V1, where the effect of spatial attention on single-unit activity is very weak [6] , [30] , [31] . This is likely due to the BOLD mechanism’s sensitivity to sub-threshold synaptic activity [24] . However, our data suggest that even presumably weak single-unit modulations can profoundly alter the distribution of population activity over a cortical region [32] , biasing neural representations in favour of the attended focus be it a location or a visual feature. In stark contrast to resolving attentional modulations, the ability to resolve V1 voxel-level orientation tuning has been largely limited to ultra-high resolution studies that only image a small volume of V1 (refs 18 , 19 ). We found that imaging with 7 T fMRI afforded a superior spatial selectivity and signal sensitivity [33] , permitting orientation tuning to be measured over a large enough volume of V1 to exclude the possibility of spatial confounds [23] . This difference in signal quality is highlighted by our finding that, in our data set the decoding accuracy of many single voxels for orthogonal orientations rivals or exceeds the accuracy of the entire V1 volume obtained at lower resolutions [21] . Single unit studies in non-human primates [7] , [12] , [13] , [34] have suggested that attention modulates responses according to a gain-like mechanism where all responses are multiplicatively increased. Such gain modulations, when combined with non-linearities such as response normalization, can explain many physiological observations [12] , [15] . Our finding that feature attention caused a simple additive increase in V1 population activity is seemingly at odds with gain-like mechanisms. However, this finding likely reflects a known discrepancy between the electrophysiology and fMRI literatures: processes which are known to evoke gain-like modulations in single units are typically associated with additive increases in the BOLD signal [24] , [35] . In our data, although additive attentional models were superior to gain-based models, the basic features of the gain terms (early facilitation in the feature domain and late suppression in the temporal domain) were completely consistent with our additive model ( Supplementary Fig. 5 ). Thus our observations, while not able to provide direct support for gain modulations at the neuronal level, are certainly consistent with such modulations underlying a broad spectrum of attentional phenomena. Consistent with the independence of spatial and featural attention [35] , [36] , we also find that independent featural and temporal attention is necessary to explain our observations. However, an interaction term is additionally required to explain the absence of net response modulation among appropriately tuned voxels after the times of likely change. This is consistent with both human event related potential [25] and monkey single unit data [8] , in which temporal expectations restrict spatial attentional modulations to behaviourally relevant periods of time. We suggest that the cumulative effect of these attentional modulations is to provide targeted feedback to neuronal populations specific for the focus of one’s attention (be it an object [37] , [38] , a location in space, a distributed visual feature) during periods of time that are most behaviourally relevant. The sensitivity of BOLD measurements to attentional modulation highlights the need for extreme caution when using imaging to study the functional architecture of cerebral cortex. Columnarly organized orientation tuning within V1 is among the most consistent phenomena in the neurophysiological literature. Its underlying basis is well-understood [17] , [39] , [40] , and efforts to resolve orientation selectivity in V1 have served as a litmus test for the resolution of columnar activity with fMRI throughout the past decade [18] , [21] . However, our results demonstrate that measurements of orientation tuning based on population activity, such as fMRI, may be heavily influenced by the observer’s mental state. In our present study, we control a subject’s attentional state and can therefore distinguish between intrinsic orientation tuning and attentional tuning changes. However, this control depended on our prior knowledge of feature selectivity in V1: namely, that neurons within V1 are strongly tuned for orientation. For areas or regions in which the underlying functional properties are less well-understood, the potential of uncontrolled behavioural factors to alter responses is a great concern. Many imaging experiments do not control for attention or attentional fluctuations, and if they do so, concentrate on spatial, but not temporal or featural, controls (for example, tasks at fixation). Even a mild, idiosyncratic preference for one of two stimuli (for example, for a face instead of an inanimate object) may cause a profound attentional modulation throughout the cortex [32] . This is particularly true for regions that are known to be modulated by subjects’ cognitive state, including association cortex and limbic structures, but as shown in our data can be a factor even at the earliest, presumably most ‘sensory’, levels of processing. Attentional modulations at such early stages can significantly bias downstream processing and allow for complex attentional changes to emerge at higher stages of processing in the visual system [15] . For example, in the case of orientation and form processing, a weighting of particular orientations could bias the sensory preferences of higher order object representations, which include that orientation, and thus be responsible for observations of ‘biased competition’ reported in single neuron studies of higher areas such as V4 (ref. 13 ). However, such a reweighting of early features would also have consequences for all the higher order visual areas receiving input from V1, including parietal areas associated with spatial and motion processing. Therefore, for tasks in which specific higher order features, such as faces or objects, are particularly behaviourally relevant it may be advantageous to directly modulate the populations that encode those higher-order features without changing all visual representations. If such higher order feature selectivity is spatially localized within a particular visual area [41] , [42] , high field imaging may be able to reveal single-voxel tuning, and attentional modulation of that tuning. Such studies could be used to directly test the hypothesis suggested by our data that all forms of attention may rely on simple linear modulations of activity that are selectively directed to task-appropriate neurons. Subjects Nine human volunteers (one author, two female volunteers, ages 20–48) participated in this study: nine performed the two Attend experiments, eight performed the No-Cue experiment and six performed the No-Rotate experiment. Data collected from one male subject were discarded due to motion artifacts. All subjects gave informed consent and the human subjects protocol was approved by the institutional review board at the University of Minnesota. Stimulus and behavioural analysis The stimulus consisted of a large continuously rotating, counter-phasing, achromatic Gabor (≈30° field of view, counter-phase frequency 2–4 Hz and rotational frequency 0.05 Hz) with a central fixation point. Use of a periodic stimulus provided enhanced statistical power to detect stimulus-evoked BOLD activity [19] , [20] . At random times, the SF of the Gabor would briefly double (from 0.5 to 1.0 cycles per degree). Subjects were required to quickly respond by button press when these SF changes occurred. To manipulate attention, subjects were notified prior to each trial (by the presentation of a 20 s static cue) whether the probability of SF changes would be uniformly distributed around all orientations (No-Cue test condition) or whether there would be a bias in the probability of SF shifts such that approximately twice as many shifts (20-fold increase in hazard function) would occur in a 45° range (full-width at half maximum (FWHM)=87.15°) centred on either 45° or 135° orientation (A45 and A135, respectively). Two subjects performed an alternative No-Cue task in which they identified a change in the colour of the centre fixation point. No difference in results was noted between subjects performing the SF-change detection and the colour-change No-Cue task, and these data are presented as one condition in this report. In a final control condition, the stimulus did not rotate but SF shifts still occurred with a predictable and sinusoidal timing (No-Rotate). Subjects received performance feedback (brief colour change) at fixation, but eye movements were not monitored and fixation was not overtly instructed. A button press within 250–750 ms of a SF shift was counted as a correctly identified target. These reaction times were averaged and used as weights in a statistical test of the second-order angular mean [43] to determine whether reaction times were uniform across all orientations. MRI acquisition Subjects viewed this stimulus via projection onto a mirror while supine in the 90 cm bore of a 7 T MR scanner, controlled by a Siemens (Erlangen, Germany) console equipped with a head gradient insert operating at up to 80 mT m −1 with a slew rate of 333 T m −1 s −1 . A half volume four-channel radio-frequency coil was used for transmission, and a nine-channel surface receive array was used for reception. We took gradient-echo (GE) echo-planar BOLD contrast functional images from a volume perpendicular to the occipital pole with a variable field of view (96 × 192 mm or 144 × 144 mm) and number of slices (25–34) but with a constant temporal and spatial resolution across subjects (repetition time (TR)=1,500 ms, echo time (TE)=20 ms, flip angle 65°, 1.5 mm isometric voxels). Retinotopic maps, when obtained, were measured using the same functional sequence over the same volume in the same session. Also in the same session and with the same hardware, high-resolution T1-weighted and proton-density anatomic images of the occipital cortex were obtained. All anatomic analyses, including volume registration, white/grey matter segmentation, and surface modelling, inflation and flattening, were performed on proton-density-normalized T1-weighted partial-volume anatomic images [44] . In MATLAB, utilizing the NIFTI Toolbox ( http://www.mathworks.com/matlabcentral/fileexchange/8797-tools-for-nifti-and-analyze-image ), raw BOLD images were visually inspected for aliasing artifacts, which were present in six subjects and manually masked. The 21st volume (the first volume after 30 s of data was discarded) of the first set of functional images collected for each subject was designated as the reference volume. All functional images from all experiments for that subject (including retinotopic mapping) were aligned via rigid-body transformation (fMRI of the Brain Software Library [45] , mcflirt function) to this reference volume, such that a given row–column–slice index referred to the same volume of cortex for all test conditions. V1/V2 ROI selection In eight subjects, standard phase-encoded retinotopic maps [46] were either collected (one 5-min scan each for polar angle and eccentricity maps, six subjects) or acquired from past experiments (two subjects). Retinotopic maps were visualized on a flattened representation of occipital cortex using FreeSurfer [47] , a V1 ROI was selected on the basis of reversals in polar angle, and this ROI was transformed into the functional image space to determine which voxels would be included for further analysis. Because the retinotopic maps were not of optimal quality (derived from a single 5-min scan instead of a typical 1 h session), we consider it likely that the V1 border was not precisely defined and that our ROI likely contains a small portion of V2 voxels. For one subject, no retinotopic data were available and anatomic volumes were manually registered to the anatomic volume of subjects with known retinotopy. This manual registration focused exclusively on aligning the calcarine sulcus, an anatomic landmark for V1. After alignment, these two subjects used the same functionally defined ROI. No difference in major results was observed between subjects with functionally and anatomically defined ROIs. All analysis of correlation between retinotopy and orientation tuning ( Supplementary Fig. 1 ) were performed exclusively on the subjects for whom retinotopic and orientation images were acquired in the same session with the same resolution over the same volume [23] . Single-voxel statistical analysis All single-voxel analysis was performed using custom software written in MATLAB, except where noted. Following motion correction, the time-series of each voxel was analyzed independently with no spatial smoothing. Not all subjects performed each control experiment; in total 51,954 voxels from V1/V2 were studied during A45/A135 (eight subjects), 45,349 voxels during No-Cue (seven subjects) and 32,226 voxels during No-Rotate (five subjects). Except when repetitions are explicitly compared, analysis was performed on concatenated data in which the time series of all repetitions of a given task were analyzed at once. Any time, data from two or more conditions are compared, the comparison is made on the same voxels from the same subjects. The first 30 s of data from each scan were discarded to eliminate start-up artifacts. We removed signal means and applied a Hamming taper to limit the effect of edge discontinuities, and a 1-dimensional, discrete Fourier transformation provided the spectral content of each voxel. From this, we estimated the phase of each voxel’s 0.05-Hz component (the frequency of stimulus rotation). This phase was adjusted by 5 s (45°) to account for the haemodynamic response latency, which was assumed to be constant in all subjects. This sinusoid plus a constant term was regressed against the raw voxel time series, where the ratio of the mean square model to the mean square model error provides an F-statistic of the goodness-of-fit of the sinusoid model. This is similar to a standard general linear model approach, except only one regressor was used. No detrending, artifact removal or other temporal filtering was performed prior to identifying modulated voxels. To limit false positives without compromising statistical power, we used the method of False Discovery Rate (FDR) to choose a critical value for our data such that only 5% of selected voxels would be false-positives [48] . A voxel with an F-statistic beyond this critical value was defined as orientation-selective, where the peak of its tuning curve, that is, orientation preference, was given via Fourier analysis and its tuning amplitude is twice the regression coefficient for the sinusoidal component. FDR-controlled data are denoted by use of a q FDR value instead of a P value in this text. Once a voxel was defined as significantly modulated, its time series was detrended by regressing out a second-order polynomial. In addition, to account for the possibility of a BOLD response to individual target events, we regressed from each voxel a predictor consisting of a target-event impulse function convolved with a canonical haemodynamic response function with a latency of 5 s. Tuning parameters of amplitude and orientation preference were then determined by finding the best-fitting sinusoid. To define a confidence interval on these tuning parameters, we computed by numerical approximation the second derivative of each voxel’s likelihood function with respect to each parameter. This derivative may be converted to a confidence interval for each tuning parameter [49] . We confirmed that our data generally met the assumptions for this form of confidence interval estimation, namely that the likelihood surface is bivariate normal at its maximum. To derive a non-parametric tuning curve for each voxel, we averaged its response to all cycles of the stimulus. These tuning curves were used to derive an estimate of the decoding accuracy (DA) for each voxel by computing the likelihood that each voxel could be explained by a sine-wave modulation at each voxel’s preferred versus anti-preferred phase. The log-likelihood ratio between preferred and anti-preferred phases ( LLR pref/anti ) provides the probability that a maximal voxel response was due to a stimulus at the preferred versus null orientation: The DA values reported in Fig. 2 were obtained by using 75% of cycle as training data to estimate the voxel’s orientation preference and the remaining 25% of cycles as validation data to obtain likelihoods relative to this orientation. For all other analyses, a single tuning curve that defined the mean of all cycles is used. To compare our orientation tuning results to previous reports, we also computed a CC at the stimulus frequency for each voxel: where F refers to the Fourier coefficient at a given frequency f . The CC is also computed after detrending and is F-distributed under the assumption of white noise [19] , [46] . To estimate the tuning width of each voxel, we required an angular distribution that might accommodate widths larger than a sine-wave to describe voxels with very poor tuning specificity. This required us to modify the standard circular Gaussian function, as the FWHM of a circular Gaussian may not be wider than a sine-wave . Our modified circular distribution consists of a square-wave with sinusoidal on- and off-ramps. It is identical to a circular Gaussian function for FWHM ≤90°, but becomes artificially wider with a flat peak for larger widths. This permitted us to estimate tuning widths from the entire range of [0°,180°). For all analyzed data, we performed a minimum of two scans (5 min each) of each condition with at least 30 min between repeats. Voxels which were significantly active during both scans had highly similar orientation preferences (A45 3.9% of voxels, A135 7.4%, No-Cue 2.8%; mode difference 0°; 95th percentile 33.6°). We concluded that our estimates of orientation tuning were reliable enough to justify concatenating all data from each condition into a single data set for all future analysis. These concatenated data gave substantially more power to detect cyclic activity. Notably, no voxel was active during two repetitions from the No-Rotate data set, leading us to conclude that these data did not contain orientation-selective information. Attentional modelling As the attentional changes observed during A45 and A135 are orthogonal ( Fig. 4 ) and independent of visual field location ( Supplementary Fig. 1 ), we combined data from the A45 and A135 to create a single Attend data set by aligning both data sets to their attended orientation. After alignment, preferred orientation and time are reported as relative to the cued orientation/time, which occurs at 0°/0 s. We then normalized the Attend and No-Cue data sets such that each voxel’s No-Cue tuning curve is defined as oscillating between 0–1. Values <0 and >1 are permitted, as these values represent real peaks above/valleys below the estimated sinusoid component. The same scaling factors were then applied to the Attend data. Thus if tuning in the Attend condition is of a larger amplitude than in the No-Cue condition, then Attend tuning curves will vary between 0 and a number >1 ( Fig. 6 ). Voxels were binned by preferred orientation and tuning curves are averaged to generate each row of the activity surfaces shown in Fig. 6 . We grouped voxels into three groups: those which exhibited orientation selectivity in all conditions (Stay-On, 7,696 voxels), those which were only selective with attention (Turn-On, n =13,876) and finally those which were only selective in the absence of attention (Turn-Off, n =5,047). Turn-Off voxels had lower tuning amplitudes (0.24% BOLD or 14% lower, t -test, 6,506 DOF, P <10 −10 ) during the No-Cue condition, and we concluded that Turn-Off voxels were predominately associated with regions whose noise precluded our ability to observe attentional effects. For all three groups of voxels, we performed a regression analysis of attended versus unattended responses to determine the potential for simple linear models to explain our data and to quantify global effects of attention. Our objective was to find the model of attention, as a function of relative preferred ( ϑ ) and stimulus (Φ) orientations that best predicts the attended responses (A45 and A135) from unattended (No-Cue) responses. First, we applied a constant phase shift to all standardized tuning curves as we found that during the Attend condition all voxels reached a peak activity ~0.5 s ( ω StayOn =0.60 s, ω TurnOn =0.65 s, ω TurnOff =0.36 s) earlier than during No-Cue conditions. Then a complete attention model, including both additive ( a ) and multiplicative ( m ) featural and temporal attention effects can be described by: where N circ is a circular Gaussian function over preferred orientation (feature) or over stimulus orientation (time) with a peak at μ and with a s.d. of σ . A F and A T are functions describing the specificity of featural and temporal modulations, respectively. Again, to accommodate attentional modulations that might be wider than π rad (FWHM>90°), we used our modified circular Gaussian as described above. Two of these parameters refer to a global non-selective attentional effect, whereby the entire surface is both multiplied ( m G ) and incremented ( a G ) by a constant. These parameters are derived by first regressing all observations across voxels and time from the Attend data set with all observations from the No-Cue data set ( Fig. 5 ), and are not allowed to covary with other model parameters. In addition, interaction parameters ( a I , m I ) test the hypothesis that these forms of attention may not be independent but rather may directly influence one another. This is an extension of an approach that has been used previously to determine the relationship between orientation preference and time during a V1 adaptation paradigm [50] : we have added the potential for additive parameters, the interaction parameters and the potential for attention functions with a FWHM> π rad. As orientation is sampled to 13 bins, each activity surface consists of 169 points, and a full model potentially consists of 13 parameters. In our data, the effects of featurally and temporally specific multiplicative gain ( m parameters) were only marginally distinguishable from the effects of the corresponding additive parameters ( a terms). Because exclusively additive models consistently performed better than exclusively gain models ( Supplementary Fig. 5 ), we set the m parameters to zero to test whether temporally and featurally specific modulations were present. Thus, because the global parameters were also set according to regression analysis on the entire data set, there were a total of three functions (featural, temporal, featural–temporal interaction) that could potentially contribute and seven parameters ( a F , a T , a I , μ F , σ F , μ T and σ T ) which needed to be evaluated and tested for significance. The maximum likelihood estimate of these parameters was found using global optimization methods ( http://www.mathworks.com/matlabcentral/fileexchange/24838-godlike-a-robust-single---multi-objective-optimizer ), and this likelihood estimate was used to compute the model’s Bayesian Information Criterion (BIC). BIC is a tool to select the most parsimonious model by imposing a penalty upon models with greater complexity. The full model BIC was compared with the BIC of submodels, in which one of these functions were removed to determine whether any smaller subset of attentional mechanisms was sufficient to explain our observed data. Such analysis revealed that all three functions were justified and the full model’s BIC was lower than that of any individual submodel. We performed a 90/10 split train/test cross-validation on this model; results from 10 repetitions gave almost identical model parameters and always provided a good explanation of the testing data ( Supplementary Fig. 3 ). To test the generalizability of this model, we separately fit the three attention functions for voxel subsets with very different attentional modulation (Stay-On, Turn-On and Turn-Off; Fig. 7 ). Approximately 86% of the variance within our activity surfaces is due to the diagonal pattern of activity that is defined by the process of generating the surface and does not reflect an attentional effect. To account for this, when reporting variance we use a measurement of ‘attentional variance’, defined as the proportion of explained variance a given model accounts for, which was not accounted for by a model with only global attention terms: where R 2 is the standard linear regression statistic commonly used to measure the amount of variance in a data set that is explained by a linear model. This adjusted attentional variance term is 0 for the global attention model, 100% for a model which perfectly recreates the observed effects of attention, and varies linearly between 0 and 100% for any model which improves upon the global attention model as measured by the R 2 metric. How to cite this article : Warren, S. et al . Featural and temporal attention selectively enhance task-appropriate representations in human primary visual cortex. Nat. Commun. 5:5643 doi: 10.1038/ncomms6643 (2014).